Tomonaga–Luttinger physics in electronic quantum circuits In one-dimensional conductors, interactions result in correlated electronic systems. At low energy, a hallmark signature of the so-called Tomonaga–Luttinger liquids is the universal conductance curve predicted in presence of an impurity. A seemingly different topic is the quantum laws of electricity, when distinct quantum conductors are assembled in a circuit. In particular, the conductances are suppressed at low energy, a phenomenon called dynamical Coulomb blockade. Here we investigate the conductance of mesoscopic circuits constituted by a short single-channel quantum conductor in series with a resistance, and demonstrate a proposed link to Tomonaga–Luttinger physics. We reformulate and establish experimentally a recently derived phenomenological expression for the conductance using a wide range of circuits, including carbon nanotube data obtained elsewhere. By confronting both conductance data and phenomenological expression with the universal Tomonaga–Luttinger conductance curve, we demonstrate experimentally the predicted mapping between dynamical Coulomb blockade and the transport across a Tomonaga–Luttinger liquid with an impurity. Despite a very large number of strongly interacting electrons, the low-lying electronic excitations in conventional bulk metals can be described as weakly interacting Fermi quasiparticles, as attested by the remarkable success of Landau’s Fermi liquid theory [1] . This picture breaks down in one-dimensional (1D) conductors, where interactions result in cooperative behaviours [2] . According to the Tomonaga-Luttinger liquid (TLL) theory [2] , [3] , [4] , [5] , [6] , the low-energy elementary excitations in 1D are collective plasmon modes, markedly different from their constitutive individual electrons. This gives rise to intriguing phenomena, such as the separation of spin and charge degrees of freedom into distinct elementary excitations propagating at different velocities [2] ; or the charge fractionalization of an injected electron [7] . Experimentally, indications of TLL physics were observed in such 1D systems as nanotubes [8] , [9] , quantum wires [10] , [11] and chains of spins [12] , [13] or atoms [14] . In addition, this physics is applicable to other many-body phenomena, including the fractional quantum Hall effect [15] , [16] , [17] , the quantum noise in 1D Bose condensates [18] and the dynamical Coulomb blockade (DCB) [19] . In the present work, we investigate experimentally the DCB conductance suppression across a quantum coherent conductor inserted in a dissipative circuit. This quantum electrodynamics phenomenon, also called zero-bias anomaly, is remarkably similar to a hallmark signature of the collective TLL physics, namely the low-energy conductance suppression in the presence of an impurity (see Fisher and Glazman [20] for a review of TLL more focused on quantum transport). In both situations, the conductance suppression originates from the granularity of charge transfers across the quantum conductor (DCB) or the impurity (TLL). Owing to Coulomb interactions, this granularity results in the possible excitation of collective electrical degrees of freedom, which impedes the charge transfers at low energy and therefore reduces the conductance. These collective degrees of freedom are the electromagnetic modes of the surrounding electrical circuit for the DCB, and the plasmon modes for a TLL. In fact, it was shown [19] that the transport across a short single-channel quantum conductor in series with a pure resistance R can be mapped rigorously onto the transport across a TLL with an impurity. Such circuits therefore provide powerful test beds for the transport across TLL systems, with many adjustable parameters including the crucial Luttinger interaction coefficient [2] , given by K =1/(1+ Re 2 / h ). Inversely, as detailed below, the mapping towards a TLL extends the theoretical understanding of DCB. To understand the quantum laws governing electrical transport in mesoscopic circuits composed of distinct quantum components, it is imperative to address the general case of the DCB for arbitrary quantum conductors. This problem remains poorly understood except in the important limit of low-transmission coherent conductors realized by tunnel junctions, which can be handled in the theory as a small perturbation to the circuit. For this class of coherent conductors embedded in a linear circuit, extensive experimental and theoretical studies have led to a good understanding [21] , [22] , [23] , [24] , [25] , [26] , [27] , [28] , [29] , [30] (see Ingold and Nazarov [31] for a pedagogical review of the theory). The tunnel limit was first overcome for relatively small conductance suppressions and low impedance environments compared with the resistance quantum . The striking prediction [32] , [33] and observation [34] are that the conductance suppression is directly proportional to the amplitude of quantum shot noise. There has also been important progress in the understanding of the regime of relatively strong conductance suppression, where the deviation to classical impedance composition laws are large (for example, Safi and Saleur [19] , Matveev et al . [35] , Flensberg [36] , Nazarov [37] , Kindermann and Nazarov [38] , Golubev et al . [39] , Zamoum et al . [40] ). In particular, the mapping of DCB to a TLL [19] opens access to the strong DCB regime for an arbitrary short single-channel quantum conductor in series with a pure resistance of arbitrary value (also see Le Hur and Li [41] and Florens et al . [42] beyond the short conductor limit). Experimentally, the strong DCB regime was recently explored for circuit impedances comparable to R q ( R =13 kΩ and 26 kΩ) (ref. 43 ); and a generalized phenomenological expression for the transmission of an arbitrary short single-channel quantum conductor embedded in a linear circuit was derived from the data (equation 1 in Parmentier et al . [43] , see also equation 1 in the present article). Does this phenomenological expression have a deeper significance? Here we show that the answer is affirmative. First, we recast equation 1 in Parmentier et al . [43] as a powerful phenomenological scaling law (equation 2) and demonstrate experimentally that it applies to a very wide range of surrounding circuits and single-channel quantum conductors. It is shown to capture the DCB data obtained for series resistances ranging from R =6–80 kΩ, and for different realizations of R (using both on-chip chromium resistance or fully transmitted quantum channels). It is also shown to apply to a very different realization of the single-channel quantum conductor from the quantum point contacts (QPCs) in a Ga(Al)As two-dimensional electron gas measured here and in Parmentier et al . [43] We demonstrate that this phenomenological expression reproduces quantitatively, essentially without fit parameters, the measurements of Finkelstein and coworkers [44] , [45] on a carbon nanotube resonant level embedded in a dissipative circuit. Second, the origin of the phenomenological expression can be traced back to the TLL collective physics. We establish this link by confronting the full universal conductance scaling curve predicted for a TLL in presence of an impurity [46] , [47] to the corresponding phenomenological scaling law for a pure series resistance R . The agreement is exact at R = R q , R << R q and, for arbitrary values of R , in the limit of a small single-channel transmission GR q <<1. At intermediate values, R ≠ R q , although relatively small deviations emerge, the proposed phenomenological scaling law is found to provide a good approximate expression for the conductance. Remarkably, the predicted mapping DCB-TLL, here extended theoretically to realistic situations in the presence of a high-frequency (for example, capacitive) cutoff, is further established by a direct comparison with the DCB conductance data. We demonstrate, with R = R q /4, a strikingly close agreement, over a broad range of conductances, with the corresponding TLL universal scaling curve computed from the exact thermodynamic Bethe ansatz solution [46] , [47] . Experimental principle The studied quantum circuits realize a tunable single-channel quantum conductor in series with an adjustable resistance. The suppression of the quantum conductor’s conductance due to DCB is extracted either by increasing the temperature or voltage (exploiting the asymptotic vanishing of DCB), or by short circuiting the series resistance in situ using an on-chip field-effect switch. A QPC of adjustable width is used as a test-bed to emulate any short single-channel quantum conductor. Experimental implementation The nano-circuits are tailored in a Ga(Al)As 2D electron gas and their conductance G ( V , T )=∂ I ( V , T )/∂ V is measured at low temperatures, in a dilution refrigerator, using standard low-frequency lock-in techniques. The samples are constituted of three basic elements ( Fig. 1 ) as described below. 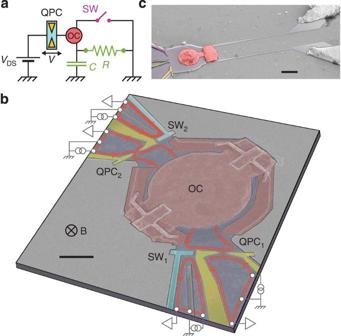Figure 1: Single electronic channel in a resistive environment. (a) Schematic circuit for the measured samples. The QPC emulates any single-channel short quantum conductor,Ris the on-chip series resistance andCis the geometrical shunt capacitance. Note thatVandVDSare, respectively, the DC voltages across the QPC and the whole circuit. (b) Colourized SEM micrograph of the sample with a series resistanceRq/nrealized by a second QPC fully transmittingnchannels. The 2D electron gas (blue) is separated in two zones by the micron-sized ohmic contact (OC). Each zone comprises a QPC (yellow split gates) and a short-circuit switch (blue gate) that allows to divert to ground the quantum Hall edge channels (red lines, here at filling factor 2) returning from the central ohmic contact. The black horizontal scale bar is 1 μm long. (c) Colourized SEM micrograph of the sample with a series resistanceR=6.3 kΩ realized by two parallel thin chromium wires visible at the right of the ohmic contact (a similar implementation was used forR=80 kΩ). The black horizontal scale bar is 2 μm long. Figure 1: Single electronic channel in a resistive environment. ( a ) Schematic circuit for the measured samples. The QPC emulates any single-channel short quantum conductor, R is the on-chip series resistance and C is the geometrical shunt capacitance. Note that V and V DS are, respectively, the DC voltages across the QPC and the whole circuit. ( b ) Colourized SEM micrograph of the sample with a series resistance R q / n realized by a second QPC fully transmitting n channels. The 2D electron gas (blue) is separated in two zones by the micron-sized ohmic contact (OC). Each zone comprises a QPC (yellow split gates) and a short-circuit switch (blue gate) that allows to divert to ground the quantum Hall edge channels (red lines, here at filling factor 2) returning from the central ohmic contact. The black horizontal scale bar is 1 μm long. ( c ) Colourized SEM micrograph of the sample with a series resistance R =6.3 kΩ realized by two parallel thin chromium wires visible at the right of the ohmic contact (a similar implementation was used for R =80 kΩ). The black horizontal scale bar is 2 μm long. Full size image First, a single-channel quantum coherent conductor characterized by its transmission probability fully adjustable between 0 and 1. It is realized by a QPC formed by field effect in the 2D electron gas using a capacitively coupled metal split gate (at the bottom right in Fig. 1b , colourized in yellow) biased at a negative voltage. The presence of well-defined plateaus at integer multiples of 1/ R q in the QPC conductance G versus split gate voltage ascertains that only one electronic quantum channel is partially open at time, with a transmission probability τ = R q G − n where n corresponds to the number of fully open quantum channels. Note that to obtain a single partially open channel, spin degeneracy was broken with a large magnetic field perpendicular to the 2D electron gas that corresponds to the integer quantum Hall effect. Consequently, the electrical current propagates along several chiral edge channels, shown as lines in Fig. 1b with arrows indicating the propagation direction. In most cases, only the outer edge channel is partially reflected/transmitted at the studied QPC. Second, a dissipative environment characterized by a linear impedance Z ( ω ). It is realized by a resistance R , made either from a thin chromium wire deposited at the sample surface ( R =6.3 and 80 kΩ, Fig. 1c ) or from a second QPC ( Fig. 1b ) set to the centre of a resistance plateau R q / n (in this case the QPC emulates a linear resistance unaffected by DCB [36] , [39] ). This resistance is in parallel with a small geometrical capacitance C ≈2 fF. The studied QPC is connected to the series resistance through a small ohmic contact (OC in Fig. 1 ). The ohmic contact is necessary to establish a connection between the surface chromium wires and the 2D electron gas buried 94 nm below the surface. In the presence of a series QPC, it also has the crucial role of an electron reservoir that separates the studied QPC and the series QPC into two distinct quantum conductors. Third, an on-chip switch to turn off DCB. The studied QPC can be isolated from the dissipative environment by diverting towards grounded electrodes the chiral edge channels that are returning from the small ohmic contact. This turns off the DCB suppression of the QPC’s conductance. In practice, it is realized using additional metal gates close to the studied QPC (for example, in Fig. 1b , the gate SW 1 is used to short circuit the dissipative environment of QPC 1 ). In the schematic representation shown in Fig. 1a , the switch is in parallel with the series resistance: when DCB is turned off, the studied QPC is directly voltage biased. Note that these extra gates allow us to characterize separately the different circuit elements, including the small ohmic contact. Test of experimental procedure in tunnel regime The experimental procedure to investigate DCB is tested by confronting the extracted conductance suppression of the QPC, set to a low-transmission probability, with the known theoretical predictions for tunnel junctions (see Ingold and Nazarov [31] ). 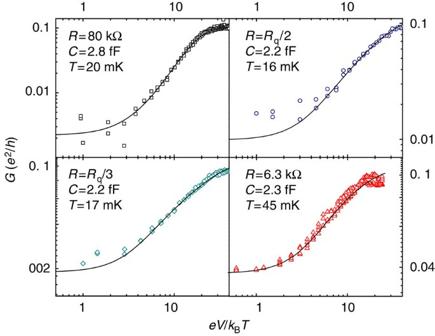Figure 2: Conductance suppression of a tunnel quantum channel in a resistive environment. Symbols: low temperature conductanceG(V,T)=∂I(V,T)/∂Vversus QPC DC voltage normalized by the temperature. Each panel corresponds to a QPC in the tunnel regime (G∞≈0.1/Rq) in series with a different on-chip resistanceR. Continuous lines: prediction of the DCB theory for tunnel junctions using the separately determined values ofR,CandTindicated in the panels. Figure 2 shows as symbols the measured QPC conductance versus DC voltage V for four different dissipative environments: two ‘macroscopic’ on-chip chromium wires ( R =6.3 kΩ and 80 kΩ) and two ‘mesoscopic’ series QPCs set to a resistance plateau ( R = R q /2 and R = R q /3). The conductance calculated using the DCB theory for tunnel junctions [31] is shown as continuous black lines. The dissipative environment in the calculation is modelled by the schematic R // C circuit shown in Fig. 1a . Note that the only adjustable parameter here is the QPC’s ‘intrinsic’ conductance G ∞ in absence of DCB, which is approximately given by the measured conductance at the highest applied voltages. The resistance R injected in the calculation is measured directly on-chip, the capacitance C corresponds to finite elements numerical simulations and the temperature T is set to that of the dilution fridge mixing chamber. Figure 2: Conductance suppression of a tunnel quantum channel in a resistive environment. Symbols: low temperature conductance G ( V , T )=∂ I ( V , T )/∂ V versus QPC DC voltage normalized by the temperature. Each panel corresponds to a QPC in the tunnel regime ( G ∞ ≈0.1/ R q ) in series with a different on-chip resistance R . Continuous lines: prediction of the DCB theory for tunnel junctions using the separately determined values of R , C and T indicated in the panels. Full size image The good agreement in the tunnel regime between data and theory validates our experimental approach. It also shows that a QPC set to a well-defined resistance plateau R = R q / n mimics a ‘macroscopic’ linear resistance [36] , [39] . 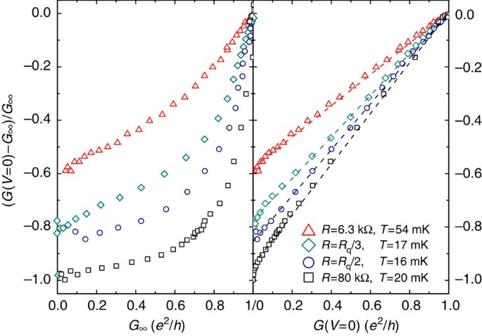Figure 3: Conductance suppression of an arbitrary quantum channel. The relative suppression of the measured zero-bias QPC conductanceG(V=0,T) with respect to ‘intrinsic’ quantum channel conductanceG∞is plotted as symbols versusG∞(left panel) andG(V=0,T) (right panel) for four series resistancesR=6.3 kΩ,Rq/3,Rq/2 and 80 kΩ. The straight dashed lines are guides for the eye. Single quantum channel conductance suppression Figure 3 shows as symbols the relative suppression of the single-channel QPC conductance measured at zero DC voltage bias and low temperature for the same four environments tested in the tunnel regime. The quantum channel is characterized by its ‘intrinsic’ conductance G ∞ , which is extracted by two methods: we either assign G ∞ to the conductance measured with the dissipative environment short circuited using the switch, or to the conductance measured at a large voltage bias where DCB corrections are small (see Supplementary Note 1 for further details). The same data are plotted in the left panel of Fig. 3 versus G ∞ , and in the right panel versus the suppressed conductance G ( V =0, T ). The non-linear dependence exhibited in the left panel shows that the prediction derived in the weak DCB framework, of a relative conductance suppression proportional to (1– R q G ∞ ) for a single channel [32] , [33] , does not hold in the strong DCB regime. Instead, we observe that the relative conductance suppression is proportional to (1– R q G ( V =0, T )) at our experimental accuracy, as seen from the linear dependence exhibited in the right panel of Fig. 3 . This result is a remarkable corroboration of the recent experimental finding in Parmentier et al . [43] , extending it to over more than one order of magnitude of the series resistance. Figure 3: Conductance suppression of an arbitrary quantum channel. The relative suppression of the measured zero-bias QPC conductance G ( V =0, T ) with respect to ‘intrinsic’ quantum channel conductance G ∞ is plotted as symbols versus G ∞ (left panel) and G ( V =0, T ) (right panel) for four series resistances R =6.3 kΩ, R q /3, R q /2 and 80 kΩ. The straight dashed lines are guides for the eye. Full size image Phenomenological expression and scaling law The experimental observation of a relative conductance suppression approximately proportional to (1– R q G ) is highly non-trivial and has strong implications. As shown in Parmentier et al . [43] ( Supplementary Note 2 ), this finding implies a phenomenological expression for the conductance G of a single channel embedded in a linear environment characterized by the impedance Z ( ω ): where is the relative conductance suppression in the tunnel regime, that can be calculated within the well-known DCB tunnel framework [31] . Note that equation 1 applies to short channels for which the energy h / τ dwell , associated with the electronic dwell time τ dwell , is larger than the other relevant energy scales (for example, eV DS , k B T , e 2 /2 C ). Indeed, even in absence of DCB, the conductance can change with the voltage and the temperature on the typical energy scale h / τ dwell (for example, owing to quantum interferences within the conductor). Moreover, a finite dwell time could result in a high-energy cutoff for the excited electromagnetic modes of the circuit, thereby reducing the overall conductance suppression due to DCB [48] . The above phenomenological expression for G requires the knowledge of the ‘intrinsic’ conductance G ∞ , which is inconvenient when this quantity is not available. This is the case for the TLL predictions, due to the presence of a high-energy cutoff in the theory, or in experimental situations such as in [44] where the conductor's conductance changes significantly at high energy even in absence of DCB. It is therefore useful to remark that the above experimental finding can be recast as a scaling law relating the transmissions τ = R q G at two different energies without involving G ∞ ( Supplementary Note 3 ): where τ 1,2 ≡ G 1,2 R q are the conductances, in units of conductance quantum, of the same single-channel quantum conductor in presence of DCB at the generator bias voltages V DS1 and V DS2 , and at the temperatures T 1 and T 2 . A direct test of the scaling is displayed Fig. 4a , where the data obtained at T =17 mK for a wide range of G ∞ , from near tunnel to near full transmission, are recast following the above scaling law with a fixed reference voltage V DS2 =9 k B T . We observe that all the data corresponding to a given series resistance R { R q /2, R q /3, R q /4} fall on top of each other, following the same black continuous line calculated with equation 2 without fit parameters. Note that we display only the data points on voltage ranges for which the separately measured energy dependency of the conductance in the absence of DCB is small (see Methods and Supplementary Note 4 ). Note also that for these series resistances, heating effects due to the voltage bias are negligible ( Supplementary Note 5 ). 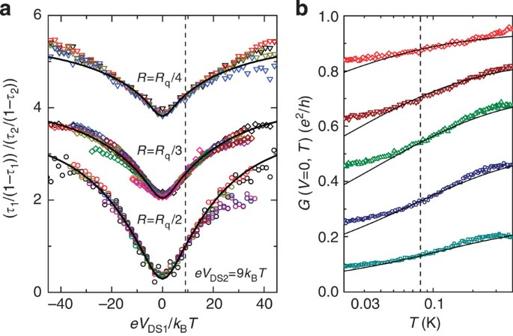Figure 4: Direct test of derived scaling law. (a) Symbols: the measured low temperature QPC transmissions (τ1,2=RqG(VDS1,DS2,T)) are recast asand plotted versusVDS1for a fixed reference voltageVDS2=9kBT. For each of the three series resistances,R=Rq/2,Rq/3 andRq/4 (corresponding data sets are shifted vertically for clarity), the QPC are tuned over a broad range ofG∞, respectively [0.06,0.95]e2/h, [0.06,0.996]e2/hand [0.25,0.85]e2/h. Continuous lines: prediction of the phenomenological scaling law equation 2 using the correspondingRandC=2.0 fF. (b) Symbols: zero-bias QPC conductance plotted versus temperature for the sample of series resistanceR=6.3 kΩ, and with five different tuning of the QPC yielding differentG∞. Continuous lines: predictions of equation 2 calculated withR=6.3 kΩ,C=2.3 fF and usingT=80 mK as the reference point. Figure 4: Direct test of derived scaling law. ( a ) Symbols: the measured low temperature QPC transmissions ( τ 1,2 = R q G ( V DS1,DS2 , T )) are recast as and plotted versus V DS1 for a fixed reference voltage V DS2 =9 k B T . For each of the three series resistances, R = R q /2, R q /3 and R q /4 (corresponding data sets are shifted vertically for clarity), the QPC are tuned over a broad range of G ∞ , respectively [0.06,0.95] e 2 / h , [0.06,0.996] e 2 / h and [0.25,0.85] e 2 / h . Continuous lines: prediction of the phenomenological scaling law equation 2 using the corresponding R and C =2.0 fF. ( b ) Symbols: zero-bias QPC conductance plotted versus temperature for the sample of series resistance R =6.3 kΩ, and with five different tuning of the QPC yielding different G ∞ . Continuous lines: predictions of equation 2 calculated with R =6.3 kΩ, C =2.3 fF and using T =80 mK as the reference point. Full size image In Fig. 4b , we make use of the scaling law for the R =6.3 kΩ series resistance’s sample by taking as a reference point the QPC conductance at T =80 mK (dashed vertical line), which is high with respect to mismatches between electronic and mixing chamber temperatures, and low regarding temperature dependencies of the ‘intrinsic’ transmission. We find that the measured conductances (symbols) plotted versus temperature obey the scaling law prediction of equation 2 (continuous lines) without any fit parameters and for a wide range of QPC tunings. Note that the discrepancies below 40 mK are possibly due to a higher electronic temperature for this set of data. Comparison with carbon nanotube resonant level The conductance suppression for a single-channel quantum conductor inserted into a dissipative environment was recently measured on a markedly different physical system than in the present work, namely a resonant level within a carbon nanotube in series with on-chip resistances [44] , [45] . The fact that the resonant peaks are wide, much more than the temperature broadening [44] , implies that the energy associated with the dwell time across the nanotube is large with respect to temperature. According to the scattering approach [49] , [50] , [51] , such a resonant level realizes at low temperatures a short single-channel quantum conductor whose apparent complexity can be encapsulated in its ‘intrinsic’ transmission probability. In Mebrahtu et al . [44] , the single-channel quantum conductor was tuned in situ by adjusting the position of the resonant level with respect to the Fermi energy and by changing the symmetry of its coupling to the two connected leads. As in the present work and in Parmentier et al . [43] , Mebrahtu et al . [44] , [45] found that the conductance through the resonant level is strongly reduced at low temperatures only when it is tuned away from full transmission (the unitary limit) . Here, we first compare the full temperature dependent conductance measured in Mebrahtu et al . [44] (symbols in Fig. 5a correspond to the data of Fig. 4a in Mebrahtu et al . [44] ) with the prediction of the phenomenological scaling law (equation 2) calculated essentially without fit parameters (continuous lines). The calculations are performed using the series resistance R =0.75 R q given in Mebrahtu et al . [44] , assuming a small parallel capacitance C =0.07 fF (there is little effect for realistic values C 0.1 fF), and using T 2 =80 mK as the reference temperature. We find a reasonable agreement between data and phenomenological scaling law (equation 2) at low enough temperatures such that the symmetric resonant level aligned with the Fermi energy (·) is perfectly transmitted. At higher temperatures, the conductance reduction in the symmetric case at the Fermi energy signals a transition towards either the sequential tunnelling regime [44] or the long dwell-time regime with energy-dependent transmissions [45] , where the phenomenological expression equation 2 for short quantum conductors does not hold. Comparisons between the phenomenological scaling law equation 2 and the other data in Mebrahtu et al . [44] , as well as those in the new preprint [45] , are available in Supplementary Note 6 . 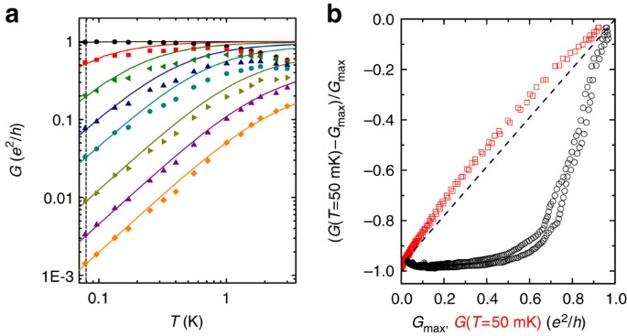Figure 5: Carbon nanotube resonant level in a resistive environment. (a) Symbols: zero-bias conductance of the carbon nanotube single-channel resonant level plotted versus temperature (data extracted fromFig. 4ain Mebrahtuet al.44), with each type of symbols corresponding to a different energy of the resonant level (tuned with a plunger gate, unity transmission corresponds to the Fermi energy44). Continuous lines: predictions calculated essentially without fit parameters with equation 2, usingR=0.75Rq,C=0.07 fF and a reference temperatureT=80 mK indicated by a dashed line. (b) The zero-bias relative conductance suppression atT=50 mK with respect to the maximum conductance (extracted from the data shown inFig. 2bof Mebrahtuet al.44) is shown as open symbols for different tunings of the resonant level position. The same data is plotted as circles versus the maximum conductanceGmaxand as squares versus the conductance atT=50 mK. Note that the appearance of two distinct curves, most visible when plotted versusGmax, corresponds to the two sets of data obtained by shifting the resonant level in opposite direction from the Fermi energy. The straight dashed line is a guide for the eye. Figure 5: Carbon nanotube resonant level in a resistive environment. ( a ) Symbols: zero-bias conductance of the carbon nanotube single-channel resonant level plotted versus temperature (data extracted from Fig. 4a in Mebrahtu et al . [44] ), with each type of symbols corresponding to a different energy of the resonant level (tuned with a plunger gate, unity transmission corresponds to the Fermi energy [44] ). Continuous lines: predictions calculated essentially without fit parameters with equation 2, using R =0.75 R q , C =0.07 fF and a reference temperature T =80 mK indicated by a dashed line. ( b ) The zero-bias relative conductance suppression at T =50 mK with respect to the maximum conductance (extracted from the data shown in Fig. 2b of Mebrahtu et al . [44] ) is shown as open symbols for different tunings of the resonant level position. The same data is plotted as circles versus the maximum conductance G max and as squares versus the conductance at T =50 mK. Note that the appearance of two distinct curves, most visible when plotted versus G max , corresponds to the two sets of data obtained by shifting the resonant level in opposite direction from the Fermi energy. The straight dashed line is a guide for the eye. Full size image To expand further on the link with the present work, we plot in Fig. 5b the relative conductance reduction at T =50 mK with respect to the maximum conductance G max measured at the same gate voltage (extracted from Fig. 2b of Mebrahtu et al . [44] ). The similarity with Fig. 3 is striking: whereas the relative conductance suppression plotted versus G max is markedly convex, it is close to a straight line when plotted as a function of G ( T =50 mK). Note that the discrepancy with a perfect linear behaviour could be attributed to difference between G max and the ‘intrinsic’ conductance G ∞ . Generalized mapping to Tomonaga–Luttinger The problem of a single-channel quantum conductor in a purely dissipative linear circuit, characterized by the series resistance R , can be mapped to that of a TLL of Luttinger interaction coefficient 1/(1+ R / R q ) (ref. 19 ). Remarkably, it can be shown that a frequency-dependent circuit impedance corresponds to the more general problem of a 1D conductor with finite-range electron-electron interactions ( Supplementary Note 7 ). In the low-energy limit, this more general model is known to reduce to a conventional TLL model with short-range interactions [6] . Similarly, we establish here that realistic circuits with a high-frequency cutoff, for example, capacitive as in Fig. 1a , can be mapped to a TLL. More specifically, we consider the impact of the next orders in the Taylor series for the real part of a frequency-dependent series impedance , where ω Z is the radius of convergence of the Taylor series expansion. As detailed in Supplementary Note 7 , the electromagnetic environment shows up in the effective bosonic action, describing the electrical transport across the quantum conductor, as an additional quadratic term proportional to , where is a bosonic field identifiable as the transferred charge. Then, by power-counting arguments, we find that the leading term is most relevant at low-energy scales. Consequently, this problem is described by the same action as for an impurity in a TLL. Note that the mapping applies provided the energy scales k B T and eV DS remain small compared with min[ ħ ω Z , ħ ω F ]. Here, ħ ω F is a TLL cutoff that delimits both the validity of the short single-channel conductor approximation (limited by the finite dwell time across the conductor and the energy barrier separating additional electronic channels) and of the linearization of the energy spectrum in the leads. Theoretical derivation of phenomenological scaling law First, for purely dissipative circuits characterized by a small series resistance Z ( ω )= R << R q but beyond the limit of weak conductance suppression, it was predicted both using a renormalization group approach [38] and exploiting the mapping to TLL [19] , [35] that the energy-dependent single-channel conductance G =τ/ R q obeys the out-of-equilibrium flow equation ( k B T << eV DS ): This equation can be integrated between the applied generator voltages V DS1 and V DS2 , which results in the same expression as the proposed phenomenological scaling law equation 2 for the corresponding limit of a purely dissipative circuit at T =0 (in which case [21] , [22] , [23] , [24] , [25] , [52] ): Remarkably, we find here, using the thermodynamic Bethe ansatz solution of the impurity problem in a TLL at k B T << eV DS (ref. 47 ), that the same flow equation 3 and, consequently, the phenomenological scaling law equation 2 are obeyed beyond the limit R << R q : as detailed in Supplementary Note 8 , we obtain the flow equation 3 exactly at R = R q within the full generalized validity domain of the mapping ( eV DS below min[ ħ ω Z , ħ ω F ]). Note that for R = R q , corresponding to a Luttinger interaction coefficient K =1/2, the same conclusions can be reached by an alternative theoretical approach referred to as the refermionization procedure [53] , [54] , [55] . We also obtain equation 3 for arbitrary values of R in the low V DS limit corresponding to small values of the suppressed transmission τ ( V DS )<<1 (even if the corresponding τ ∞ is close to unity). Comparison TLL-phenomenological scaling law Now that the validity of the proposed phenomenological scaling law (equation 2) is theoretically established in the three different limits τ ( V DS )<<1, R << R q and R = R q , we confront its predictions at intermediate values of R with numerical evaluations of the exact TLL universal conductance curve. In Fig. 6 , we display such a comparison for the intermediate series resistance R = R q /4 on the full range of single-channel conductances. The out-of-equilibrium ( k B T << eV DS ) TLL prediction for the conductance in the presence of an impurity follows a universal scaling curve G TLL ( V DS / V B ), with V B a scaling voltage encapsulating the impurity potential. As detailed in Supplementary Note 8 , this conductance can be numerically computed using the exact thermodynamic Bethe ansatz solution [46] , [47] (red dashed line in Fig. 6 ). Although the conductance curve depends on the TLL interaction coefficient K =1/(1+ R / R q ), it is universal in the sense that the same curve applies for an arbitrary local impurity. Note that there is no universal relation between V B and the ‘intrinsic’ transmission probability τ ∞ of the corresponding DCB problem. For instance, such a relation would depend on the specific high-frequency behaviour of Z ( ω ). The conductance predicted by the phenomenological scaling law equation 2 is shown as a continuous black line in Fig. 6 . In the corresponding limit of a pure series resistance Z ( ω )= R q /4 at k B T << eV DS , it takes the simple analytical form given by equation 4. The single reference point used in the phenomenological scaling law is the TLL conductance prediction at a very low voltage bias V DSref / V B =0.0005, where it is theoretically established that both predictions match. Note that there is no need to fix the scaling voltage V B here, as only the voltage ratio with respect to V DSref is needed in equation 4. 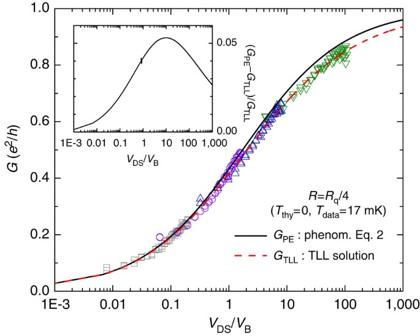Figure 6: Comparison TLL universal conductance curve-phenomenological scaling law-data forR=Rq/4, beyond the theoretically established validity of the phenomenological scaling law. Red dashed line: universal conductance scaling curveGTLL(VDS/VB) computed from the TLL thermodynamic Bethe ansatz solution atT=0 (refs46,47) (Supplementary Note 8). Black straight line: conductanceGPEpredicted by the phenomenological scaling law given by equation 4 for a pure series resistance atT=0. The full conductance curveGPE(VDS/VB) was calculated using the single reference pointGPE=GTLLatVDSref/VB=0.0005. Symbols: four data sets measured atT=17 mK in the presence of a series resistanceR=Rq/4. The corresponding scaling voltagesVB=330 μV (open squares), 40 μV (open circles), 8 μV (open upright triangles) and 0.6 μV (open downward triangles) are obtained by matchingGTLL(VDSref/VB) with the conductance measured at the reference pointVDSref=9kBT13 μV (note that a better agreement data–phenomenological scaling law would have been obtained using insteadGPE(VDSref/VB)). Inset: relative deviations of the conductance calculated using the phenomenological expression equation 2 with respect to the universal conductance scaling curve (GPE−GTLL)/GTLL. Figure 6: Comparison TLL universal conductance curve-phenomenological scaling law-data for R = R q /4, beyond the theoretically established validity of the phenomenological scaling law. Red dashed line: universal conductance scaling curve G TLL ( V DS / V B ) computed from the TLL thermodynamic Bethe ansatz solution at T =0 (refs 46 , 47 ) ( Supplementary Note 8 ). Black straight line: conductance G PE predicted by the phenomenological scaling law given by equation 4 for a pure series resistance at T =0. The full conductance curve G PE ( V DS / V B ) was calculated using the single reference point G PE = G TLL at V DSref / V B =0.0005. Symbols: four data sets measured at T =17 mK in the presence of a series resistance R = R q /4. The corresponding scaling voltages V B =330 μV (open squares), 40 μV (open circles), 8 μV (open upright triangles) and 0.6 μV (open downward triangles) are obtained by matching G TLL ( V DSref / V B ) with the conductance measured at the reference point V DSref =9 k B T 13 μV (note that a better agreement data–phenomenological scaling law would have been obtained using instead G PE ( V DSref / V B )). Inset: relative deviations of the conductance calculated using the phenomenological expression equation 2 with respect to the universal conductance scaling curve ( G PE − G TLL )/ G TLL . Full size image We find a good quantitative agreement between TLL and phenomenological scaling law predictions on the full range of bias voltages and conductances, with relatively small deviations appearing at large bias voltages ( 5%, see inset of Fig. 6 ). This good agreement corroborates the predicted mapping DCB-TLL. It is noteworthy that the phenomenological scaling law equation 2 encompasses arbitrary linear circuit impedances Z ( ω ), beyond the limit of a series resistance , suggesting a possible generalization of the TLL predictions. Experimental test of predicted mapping TLL-DCB The most straightforward experimental test consists in the direct comparison of the conductance data with the universal conductance scaling curve G TLL ( V DS / V B ). Figure 6 displays such a comparison for the series resistance R = R q /4. Four data sets of the conductance measured at T =17 mK, each corresponding to a different tuning of the QPC embedded in the same R = R q /4 environment, are shown as symbols. For each data set, the value of V B is fixed by matching the measured conductance at a single arbitrary reference voltage V DSref =9 k B T 13 μV with the TLL prediction for the conductance G TLL ( V DSref / V B ). This gives V B =330 μV, 40 μV, 8 μV and 0.6 μV. Note first that the lowest voltage in each data set corresponds to ~3 k B T / e , thereby minimizing the effect of the finite experimental temperature. Note also that the highest voltage in each data set V DS ≈65 μV is smaller than h / eRC ≈300 μV, which limits the contribution of the experimental short-circuit capacitance C 2 pF to the series impedance . We observe that the conductance data closely obey the TLL predictions over the full range of single-channel conductances and over four order of magnitudes of V DS / V B . This observation constitutes a direct experimental demonstration that the transport across a single-channel quantum conductor embedded in a dissipative environment can be mapped onto collective Tomonaga–Luttinger liquid behaviours. The present work is at the crossroad of two seemingly distinct phenomena namely, on the one hand, the Tomonaga–Luttinger physics of interacting 1D conductors and, on the other hand, the different set of quantum laws of electricity when distinct quantum coherent conductors are assembled into a circuit. By advancing and confronting both the experimental and theoretical aspects, we have established the predicted link between these two phenomena for the basic class of mesoscopic circuits constituted by a short single-channel quantum conductor in series with a linear resistance. This opens the path to using electronic circuits as test beds for Luttinger physics, and also advances our understanding of the quantum laws of electricity through the powerful TLL theoretical framework. In particular, important insight may be obtained in the investigation of the direct link between suppressed conductance and quantum shot noise, that is expected to hold even in the regime of strong conductance suppression [19] , [38] (see also Supplementary Note 9 ). An important outcome of the present work is that we strongly consolidate, delimit the validity, and grasp the significance of the generalized phenomenological expression equation 1 for the conductance of an arbitrary short quantum channel in a linear environment. From an experimental standpoint, its validity is demonstrated for a wide range of circuit impedances, and is found in good agreement with the data of Mebrahtu et al . [44] , [45] obtained on a different physical system, a carbon nanotube resonant level. From a theoretical standpoint, the equivalent scaling law equation 2 is derived for the suppressed conductance in various limits, in particular for a series resistance R = R q . We also find that relatively small deviations exist in intermediate regimes. These results are not only of fundamental importance; the knowledge of the different quantum laws of electricity with coherent conductors has also direct implications for the quantum engineering of future nanoelectronic devices. Measured samples The samples are nanostructured by standard e-beam lithography in a 94-nm-deep GaAs/Ga(Al)As 2D electron gas of density 2.5 × 10 15 m −2 and mobility 55 m 2 V −1 s −1 . Experimental setup The measurements were performed in a dilution refrigerator with a base temperature of T =16 mK. All measurement lines were filtered by commercial π-filters at the top of the cryostat. At low temperature, the lines were carefully filtered and thermalized by arranging them as 1 m-long resistive twisted pairs (300 Ω m −1 ) inserted inside 260 μm inner diameter CuNi tubes, which were tightly wrapped around a copper plate screwed to the mixing chamber. The samples were further protected from spurious high-energy photons by two shields, both at the mixing chamber temperature. Measurement techniques The differential conductance measurements were performed using standard lock-in techniques at frequencies below 100 Hz. To avoid sample heating, the AC excitation voltages across the sample were smaller than k B T / e . The sample was current biased by a voltage source in series with a 10 MΩ or 100 MΩ polarization resistance. The bias current applied to the drain was converted on-chip into a fixed V DS , independent of the QPC conductance, by taking advantage of the well-defined quantum Hall resistance to ground of the drain electrode ( R q / n at filling factor ν = n ). Similarly, the current across each component (QPCs, switches) is obtained by converting the voltage measured with the amplifiers represented as triangles in Fig. 1 using the R q / n quantum Hall resistance. The conductances of the QPC, switch and series chromium wires or series QPC were obtained separately by three point measurements. For all the samples, we used cold grounds directly connected to the mixing chamber of the dilution refrigerator. Test of the small ohmic contacts The electrical connection between the small ohmic contact (labelled OC in Fig. 1b ) and the buried 2D electron gas was tested with both the QPCs and the switches set in the middle of the very large and robust conductance plateau G =2/ R q . Assuming that the two outer edge channels are fully transmitted across QPCs and switches, and that the inner channels are fully reflected, we find for all samples that the reflection of each of the two outer edge channels on the small ohmic contact is smaller than 0.01. Energy dependences of ‘intrinsic’ conductance A coherent conductor may present energy dependences in its ‘intrinsic’ conductance G ∞ associated with, for example, a finite dwell time. In the case of QPCs, these often result from nearby defects. These energy dependences add up with the DCB energy dependence, which makes the extraction of the DCB signal as a function of voltage and temperature more difficult. In Supplementary Note 4 , we illustrate the energy behaviour of the QPCs with the electromagnetic environment short circuited and explain how we deal with the energy dependences of G ∞ in the present work. How to cite this article: Jezouin, S. et al . Tomonaga–Luttinger physics in electronic quantum circuits. Nat. Commun. 4:1802 doi: 10.1038/ncomms2810 (2013).